A network of genes connects polyglutamine toxicity to ploidy control in yeast Neurodegeneration is linked to protein aggregation in several human disorders. In Huntington’s disease, the length of a polyglutamine stretch in Huntingtin is correlated to neuronal death. Here we utilize a model based on glutamine stretches of 0, 30 or 56 residues in Saccharomyces cerevisiae to understand how such toxic proteins interfere with cellular physiology. A toxicity-mimicking cytostatic effect is evident from compromised colony formation upon expression of polyglutamines. Interestingly, diploid cells are insensitive to polyglutamines and haploid cells can escape cytostasis by hyperploidization. Using a genome-wide screen for genes required to obtain the cytostatic effect, we identify a network related to the budding process and cellular division. We observe a striking mislocalization of the septins Cdc10 and Shs1 in cells arrested by polyglutamines, suggesting that the septin ring may be a pivotal structure connecting polyglutamine toxicity and ploidy. Protein misfolding and aggregation are initial steps towards certain neuropathies. For Huntington’s disease and related pathologies, the extension of CAG repeats, as in the first exon of the huntingtin (Htt) gene HTT , translate into extended polyglutamine (polyQ) stretches and render the affected proteins aggregation-prone [1] , [2] , [3] . The threshold for the transition from a non-pathogenic extension to dominant pathogenicity was shown to be 35–45 glutamine residues [4] , [5] , [6] . Understanding the relation between glutamine extension and cellular toxicity is essential to understand the aetiology of such disorders. Different models have been established to analyse aggregate formation and toxicity in living cells [7] , [8] , [9] , [10] , [11] , [12] , [13] . Overexpressing Htt variants resulted in aggregate formation and death of cultured mammalian cells [14] . Similarly, amino-terminal fragments of the HTT gene with long stretches of polyQ compromised growth [15] by compromising the translational machinery in yeast [16] . This system’s toxicity appeared to be dependent on the folding status of endogenous prion proteins like Rnq1 (ref. 17 ). Although elaborate machineries that control aggregation exist [18] , proteotoxicity arises via pathways that are still not entirely understood. Studies investigating the cell biology of protein aggregation in yeast further uncovered that the controlled asymmetric inheritance of aggregates is dependent on the polarisome and the cytoskeleton [19] , [20] . Moreover, different types of misfolded proteins have been shown to be recruited to specific quality control compartments: the juxtanuclear quality control compartment or perivacuolar foci [21] . In respect to toxicity, a recent study indicated that the cytotoxic effect of aggregation-prone proteins is likely generated by the sequestration of essential cellular hub proteins into aggregates [22] . To probe the toxicity of polyQ proteins in baker’s yeast, we established a system characterized by a slow growth phenotype. We identify pathways that generate polyQ-induced cytostasis and perceive a surprising connection between proteotoxicity and the ploidy state of the cell. A Q56 polyQ stretch inhibits growth of yeast cells To study aggregation in yeast, we designed polyQ proteins that are close to the human toxicity threshold. Zero, 30 or 56 glutamine residues were fused to the yellow fluorescent protein (Q 0 -YFP, Q 30 -YFP and Q 56 -YFP) and the encoding plasmids pQ0, pQ30 and pQ56 were transformed into wild-type (WT) MAT a yeast cells. A homogeneous colony pattern developed when transformed with pQ0 and pQ30. Contrarily, transformation with pQ56 yielded inhomogeneous patterns, comprising 95% small colonies, 4% intermediate size colonies and 1% large colonies ( Fig. 1a ). To estimate the growth potential of cells, individual colonies were replated. Colonies transformed with pQ0 and pQ30 contained about 1200 colony forming units (CFUs) per 1 × 10 4 cells. A similar number of CFUs was obtained for the few large colonies on pQ56 plates. The predominant small colonies transgenic for pQ56, however, contained only between 1 and 15 CFUs per 1 × 10 4 plated cells, indicating that cytostasis persists for about 99% of the cells forming a colony. We termed this phenotype polyQ-induced cellular arrest ( pica ). 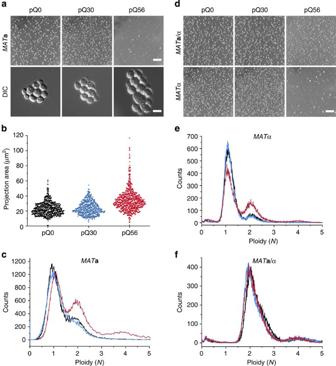Figure 1: A population-based growth phenotype in yeast. (a, upper row) WT haploidMATayeast exhibits apicaphenotype, which is only observable after transformation with pQ56 (right column) but not in control transformations with pQ0 (left column) and pQ30 (middle column). Size differences between Q56-YFP expressing yeast and the Q0and Q30controls become obvious in differential interference contrast (DIC) microscopy (lower row). The scale bar represents 10 mm in the upper row and 5 μm in the lower row. (b) Analysing the cellular cross-section area for the predominant colony type, pQ56-transformants exhibit a subpopulation of cells of a larger size (n=740,n=659 andn=769 for pQ0, pQ30 and pQ56, respectively;Supplementary Fig. 3for further biological replicates). (c) FACS analysis of WTMATareveals a higher incidence of 2Nand 4Ncells in response to pQ56 transformation (red) compared with pQ0 (black) and pQ30 (blue). (d) Transforming diploid WTMATa/α and WTMATα shows that thepicaphenotype is conserved in theMATα genetic background but absent in the diploid strain. (e) In FACS, WTMATα still exhibits a mainly haploid state and an enrichment in 2Nand 4Nstates after pQ56 transformation. (f) The diplod WTMATa/α strain transformed with pQ0 (black), pQ30 (blue) and pQ56 (red), however, shows an equal shift to the 2Nand 4Npositions for all polyQ constructs. Figure 1: A population-based growth phenotype in yeast. ( a , upper row) WT haploid MAT a yeast exhibits a pica phenotype, which is only observable after transformation with pQ56 (right column) but not in control transformations with pQ0 (left column) and pQ30 (middle column). Size differences between Q 56 -YFP expressing yeast and the Q 0 and Q 30 controls become obvious in differential interference contrast (DIC) microscopy (lower row). The scale bar represents 10 mm in the upper row and 5 μm in the lower row. ( b ) Analysing the cellular cross-section area for the predominant colony type, pQ56-transformants exhibit a subpopulation of cells of a larger size ( n =740, n =659 and n =769 for pQ0, pQ30 and pQ56, respectively; Supplementary Fig. 3 for further biological replicates). ( c ) FACS analysis of WT MAT a reveals a higher incidence of 2 N and 4 N cells in response to pQ56 transformation (red) compared with pQ0 (black) and pQ30 (blue). ( d ) Transforming diploid WT MAT a /α and WT MAT α shows that the pica phenotype is conserved in the MAT α genetic background but absent in the diploid strain. ( e ) In FACS, WT MAT α still exhibits a mainly haploid state and an enrichment in 2 N and 4 N states after pQ56 transformation. ( f ) The diplod WT MAT a /α strain transformed with pQ0 (black), pQ30 (blue) and pQ56 (red), however, shows an equal shift to the 2 N and 4 N positions for all polyQ constructs. Full size image Fluorescence microscopy of the transformant plates revealed that only a subset of the few large colonies transformed with pQ56 exhibited fluorescence levels comparable to the control colonies producing Q 30 -YFP or Q 0 -YFP. The Q 56 -YFP level in pica colonies instead was much lower ( Supplementary Fig. S1 ). This was confirmed by immunogenic detection of the YFP fusion proteins in cell lysates ( Supplementary Fig. S2 ). Fluorescence microscopy revealed a differential pattern of subcellular distribution of the polyQ proteins. No fluorescent foci were present in cells transformed with pQ0, but Q 30 -YFP and Q 56 -YFP-producing cells exhibited aggregate formation of different qualities and at a very low incidence for pQ56 ( Supplementary Fig. S1 ). Based on these data we assume that Q 0 -YFP and Q 30 -YFP are not cytostatic, while Q 56 -YFP, despite low cytosolic levels, is highly cytostatic. Higher ploidy leads to polyQ resistance Impaired growth may lead to morphological phenotypes. Consequently, we studied the morphology of transformants and realized that cells from small colonies of pQ56 plates appeared enlarged compared with controls ( Fig. 1a ). More detailed analysis of cell sizes confirmed that pica colonies contain more large cells than pQ0- and pQ30-transformed colonies ( Fig. 1b and Supplementary Fig. 3 ). As alterations to the cell cycle may result in enlarged cells, we employed fluorescence activated cell sorting (FACS) to measure cellular DNA content. FACS analysis showed that histograms from cells transgenic for pQ0 and pQ30 are almost superimposable: both represent haploid cells cycling between states of one genome copy (1 N ) and two genome copies (2 N ). Yeast cells from pQ56 transgenic plates instead contain more 2 N cells and a small fraction of cells in a 4 N state ( Fig. 1c ), implying that the presence of Q 56 -YFP may lead to an enrichment of cells with a higher content of DNA. As some large colonies on pQ56 plates seem to be able to overcome growth inhibition and are even brightly fluorescent, we isolated plasmids from such colonies and sequenced the polyQ encoding region to determine the actual length of the polyQ stretch. Many large colonies, in particular those with high fluorescence levels, showed a dramatically shortened polyQ stretch, while others grew despite stretches longer than 50 glutamines ( Supplementary Table S1 ). We also used FACS to study these large survivor colonies. The resistant colonies containing stretches of over 50 glutamines exhibited a ≥2 N signature in FACS measurements ( Supplementary Table S1 , Supplementary Fig. S4 ). This finding indicates that large colonies on pQ56 transformant plates are able to grow normally by an accumulation of another chromosome set. To test whether diploid strains in general are not sensitive to Q 56 -YFP, we transformed the diploid isogenic WT MAT a /α strain. The pica phenotype was abolished ( Fig. 1d ). However, the corresponding WT MAT α haploid strain remained pica ( Fig. 1d ). We also analysed homozygous WT diploid strains of MAT a/a and MAT α/α genotypes [23] in order to test, whether heterozygosity at the mating type locus causes the resistance towards pica . Both are insensitive towards pQ56 ( Supplementary Fig. S5 ), confirming that Q 56 -YFP is well tolerated also in yeasts containing two identical chromosome sets, while haploid cells suffer from the cytotoxicity exerted by this protein’s presence. These data suggest that the acquisition of a diploid state may lead to the appearance of cells of higher ploidy within slowly growing colonies. The low incidence of resistant clones implies nevertheless, that growth-promoting conversions occur rarely, although enlargement is frequent. A genome-wide screen reveals enhancers of cytostasis As the pica phenotype can be rescued spontaneously, we screened all 5130 haploid knockouts of the Saccharomyces Genome Deletion Project [24] in the MAT a background to identify genes involved in mediating the cytostatic effect of Q 56 -YFP ( Fig. 2a ). All strains were transformed with pQ56 plasmid and their colony growth pattern was evaluated individually. Knockout strains showing more homogeneous growth than the WT strain were retained. These strains were then rescreened, yielding 68 knockout strains, which reliably rescued pica ( Fig. 2b ). As MAT a /α diploids would yield positive results, we assessed the mating type status of each strain by PCR. Thirty strains turned out to be MAT a /α ( Supplementary Table S2 ), while the others were only positive for MAT a as to be expected for library strains. 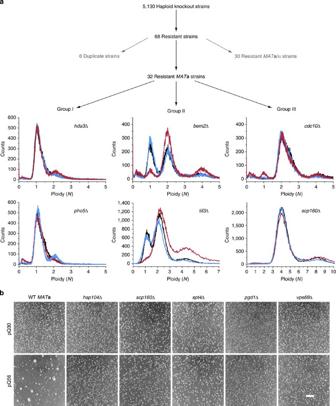Figure 2: A summary of the screen for genes enhancing thepicaphenotype of Q56-YFP. (a) All available 5130 haploid non-essential knockouts in theMATabackground were transformed with pQ56 plasmid and their colony growth pattern was evaluated individually. Sixty-eight strains were found to reduce thepicaphenotype of pQ56. Six genes were targeted by two strains in the library, 30 diploidMATa/α strains were excluded, leaving 32 strains after the screen. By FACS analysis, the enhancers ofpicawere classified into three groups, based on their behaviour in response to pQ0 (black), pQ30 (blue) or pQ56 (red). For each group, the results for two representative strains are shown. (b) Representative images of deletion strains that are resistant to Q56-YFP show that in many cases the pQ56-inducedpicaphenotype (lower row, left column) disappears and normal growth in comparison with pQ30 (upper row) is restored as shown for the strainshsp104Δ,scp160Δ,spt4Δ,pgd1Δandvps69Δ. Scale bar represents 10 mm. Figure 2: A summary of the screen for genes enhancing the pica phenotype of Q56-YFP. ( a ) All available 5130 haploid non-essential knockouts in the MAT a background were transformed with pQ56 plasmid and their colony growth pattern was evaluated individually. Sixty-eight strains were found to reduce the pica phenotype of pQ56. Six genes were targeted by two strains in the library, 30 diploid MAT a /α strains were excluded, leaving 32 strains after the screen. By FACS analysis, the enhancers of pica were classified into three groups, based on their behaviour in response to pQ0 (black), pQ30 (blue) or pQ56 (red). For each group, the results for two representative strains are shown. ( b ) Representative images of deletion strains that are resistant to Q 56 -YFP show that in many cases the pQ56-induced pica phenotype (lower row, left column) disappears and normal growth in comparison with pQ30 (upper row) is restored as shown for the strains hsp104Δ , scp160Δ , spt4Δ , pgd1Δ and vps69Δ . Scale bar represents 10 mm. Full size image The annotated function of the final set of genes suggests transcription, translation and budding/cellular division being involved in the generation of toxicity ( Fig. 3 , Supplementary Table S3 ). The proteins Med2, Rox3, Pgd1 and Sin4 are subunits of the mediator complex, regulating RNA-polymerase II transcription [25] , while Spt4 is a general regulator of RNA-polymerase and pre-mRNA processing [26] . The proteins Scp160, Eap1, Asc1 and Bfr1 are part of the SESA (Smy2, Eap1, Scp160 and Asc1) network, coordinating spindle pole duplication by regulating the transcription of kinetochore-specific mRNA, hence linking translation to nuclear division [27] . Bem2 is known to be crucial to determine the future site of bud emergence and to allow the deposition of the septin ring. Cdc10 is part of this structure [28] . Hsl7, as well as Hof1 and Cyk3, functionally interact with the septin ring during budding [29] , [30] . The ring has previously been reported to serve as a signalling scaffold during bud maturation [31] . In this context, it is interesting to note, that the disaggregase Hsp104 (ref. 32 ) cooperates with Hof1 and the actin network to maintain the asymmetric distribution specifically of damaged or aggregated proteins between the mother and daughter cell [19] , [33] . 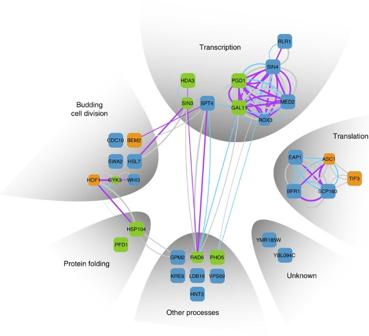Figure 3: A network of genes is required to obtain thepicaphenotype of Q56-YFP. The genes uncovered in the genome-wide screen are depicted as squares. The size of each square corresponds to the quality of the hit in respect to the pQ56 system. Square colour represents group association (green: Group I, orange: Group II, blue: Group III). Known interactions of the genes are represented by edges. The width of the edges correlates to the confidence level, the colour reflects the type of evidence (purple: physical interaction, blue: text mining, grey: other method). The genes were clustered according to their annotated biological process contribution (Supplementary Table S3for further details). Figure 3: A network of genes is required to obtain the pica phenotype of Q 56 -YFP. The genes uncovered in the genome-wide screen are depicted as squares. The size of each square corresponds to the quality of the hit in respect to the pQ56 system. Square colour represents group association (green: Group I, orange: Group II, blue: Group III). Known interactions of the genes are represented by edges. The width of the edges correlates to the confidence level, the colour reflects the type of evidence (purple: physical interaction, blue: text mining, grey: other method). The genes were clustered according to their annotated biological process contribution ( Supplementary Table S3 for further details). Full size image Several of the genes identified have been implicated in the control of chromosome number and the generation of higher ploidy. Having previously established a link between cytostasis and the number of chromosome sets, we deployed FACS analysis to test whether the strains we found are de facto haploid. Based on fluorescence histograms, the strains were categorized into three groups (I–III, Fig. 2a , Supplementary Table S3 ). Group I members behave WT-like. They gain a minor population with a ≥2 N signature upon pQ56 transformation. Group II has a haploid-typic 1 N /2 N cycling behaviour, if transgenic for pQ0 and pQ30. However, upon transformation with pQ56, the 1 N peak is lost and the population mainly consists of cells of a 2 N state and higher ploidy. Group III holds knockout strains with more than one set of chromosomes, even if transformed with the non-toxic pQ0 and pQ30 controls. As such, scp160Δ is annotated to accumulate additional genome copies and was appropriately sorted into this group [34] . It is tempting to speculate that the genes identified, which are connected to the budding process, warrant the maintenance of the haploid status in a pathway that becomes growth inhibiting in the presence of Q 56 -YFP. Genetic manipulation of this network enables cells to overcome the pica phenotype. Would the genes we found also be required for the toxicity of a previously described aggregation model based on a Htt fragment [15] ? Using this system in analogy to our assays, HttQ103 transformants showed no growth—despite sporadic large colonies—while a homogeneous colony pattern developed for the HttQ25 control ( Supplementary Fig. S6 ). Of the 38 knockout strains obtained in our screen, 28 strains also reduce HttQ103 toxicity, but not necessarily to a full extent ( Supplementary Table S3 ). This implies that most of the genes uncovered are involved in the generation of the cytostatic effect exerted by polyQ proteins, independent of the system used and its protein context. To understand whether rescue by higher ploidy may also be common to both systems, we transformed diploid and tetraploid strains. MAT a / a or MAT α/α exhibit incomplete rescue, whereas the tetraploid strains PY5006 ( MAT a / a / a / a) and PY5007 ( MAT α/α/α/α) [23] were fully resistant to HttQ103 toxicity ( Supplementary Fig. S7 ). Consequently, polyploidy is a shared mechanism of resistance for the HttQ103 and the Q 56 -YFP model systems. Endogenous prion marginally influences the pQ56 system In particular Hsp104, which is part of our Group I, has long been known to be a major player in aggregation and prion-related processes in yeast [32] , [35] . Guanidine hydrochloride (GdnHCl) is a known inhibitor of the disaggregase Hsp104 and a prion curing agent [36] . We thus tested the effect of this agent on our system. Plates containing 4 mM GdnHCl strongly reduce the pica phenotype ( Supplementary Fig. S8a ) and in FACS analysis GdnHCl induced rescue is indistinguishable from the deletion of HSP104 ( Supplementary Fig. S8b,c ). Previous studies had shown that the toxicity of the Htt-derived polyQ construct is dependent on the state of endogenous prion proteins in yeast. Specifically, the protein Rnq1 had been described to be required in its [ PIN + ] prion state to obtain HttQ103 toxicity [17] , [37] . Surprisingly, we did not recover RNQ1 in our screen. We thus wanted to know, whether toxicity is prion-mediated. In this case, the deletion of RNQ1 should abolish the toxicity of the pQ56 system. We confirmed that in the absence of RNQ1 , the phenotype of the HttQ103 system is fully abolished ( Supplementary Fig. S9 ). However, for pQ56, only a partial rescue of pica is observable, resulting in a reproducible increase in large colonies. We tested, whether this effect is due to different subpopulations in the bulk cultures derived from glycerol stocks, by picking individual clones and testing them separately. Of 15 separate clones transformed, 2 abolished the phenotype in both systems. However, 13 clones exhibited a pica phenotype for pQ56 but abolished the toxicity of HttQ103. This result indicates, that HttQ103 and Q 56 -YFP differ in respect to their dependence on the prion state of Rnq1. If the maintenance of the pica phenotype was due to another protein being in its prion state, a complete loss of endogenous proteins in prion conformation should abolish pica . This ‘prion curing’ can be achieved by the sequential passage of a strain on a medium containing 4 mM GdnHCl and has been previously applied as a control for prion effects [38] . Prion curing was performed to compare the HttQ103 system to the pQ56 system. The cured MAT a WT prion-negative strain showed no phenotype of HttQ103, but exhibited an unchanged pica phenotype for pQ56 ( Supplementary Fig. S9 ). This result confirms that the toxicity of pQ56 is only weakly correlated with the prion state of the cell. Loss of HSP104 and PHO5 changes behaviour of Q 56 -YFP To understand the resistance of Group I hits, we initially analysed the amount of Q 56 -YFP in Group I strains. All knockouts contain levels of polyQ protein that roughly equal WT levels ( Fig. 4a ). They all synthesize a long polyQ species also present in the WT strain, confirming that the polypeptide of toxic length is produced at similar amounts. However, the expression of the toxic transgene is strongly increased in the strains hsp104Δ , pho5Δ , and in the presence of GdnHCl. It has been shown before, that polyQ toxicity may be altered by the oligomerization state of polyQ proteins [39] . To clarify, whether changes to the molecular oligomerization pattern of Q 56 -YFP are correlated with the loss of the pica phenotype, we performed native agarose gel electrophoresis [39] . In lysates of pho5Δ , hsp104Δ , and GdnHCl-treated WT, a gel-permeable but apparently very large species was present ( Fig. 4b ). 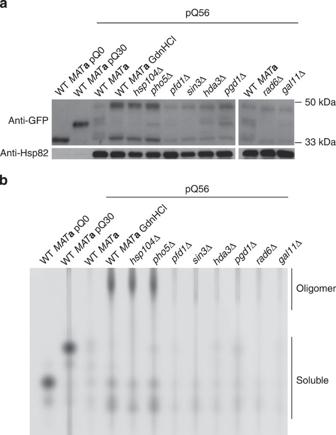Figure 4: Q56-YFP levels increase and its molecular state changes when Hsp104 or Pho5 are lost. (a) Western blotting against GFP reveals that the expression of the Q56-YFP protein is not diminished in any of the Group I knockout strains. Instead, expression is increased in the GdnHCl-treated WTMATastrain and the strains with deletions ofHSP104andPHO5. Hsp82 was used as a loading control. (b) Native agarose gel electrophoresis reveals oligomeric forms of Q56-YFP upon the addition of GdnHCl and the deletion ofHSP104orPHO5. This is not the case when other genes of Group I are deleted. In both panels, the lysates from WTMATatransformed with pQ0 and pQ30 were diluted 15-fold to enable simultaneous detection of all lysates on the same gel and western blot. Figure 4: Q 56 -YFP levels increase and its molecular state changes when Hsp104 or Pho5 are lost. ( a ) Western blotting against GFP reveals that the expression of the Q 56 -YFP protein is not diminished in any of the Group I knockout strains. Instead, expression is increased in the GdnHCl-treated WT MAT a strain and the strains with deletions of HSP104 and PHO5 . Hsp82 was used as a loading control. ( b ) Native agarose gel electrophoresis reveals oligomeric forms of Q 56 -YFP upon the addition of GdnHCl and the deletion of HSP104 or PHO5 . This is not the case when other genes of Group I are deleted. In both panels, the lysates from WT MAT a transformed with pQ0 and pQ30 were diluted 15-fold to enable simultaneous detection of all lysates on the same gel and western blot. Full size image We wondered, whether this change in oligomerization is also reflected on the level of cellular aggregate formation. As shown above, cells expressing Q 0 -YFP exhibit a homogeneous distribution of fluorescence throughout the cytoplasm. This is not the case for Q 30 -YFP and Q 56 -YFP. Both can form visible aggregate-like structures. For Q 30 -YFP these sometimes have a fibrous appearance ( Supplementary Fig. S10 ). Most Q 56 -YFP-producing cells did not show visible aggregate-like structures potentially due to low expression levels ( Fig. 4a ). In case we observed aggregates, they exhibited punctate or spherical structures ( Supplementary Fig. S10 ). While for all other Group I hits this pattern was similar, hsp104Δ and pho5Δ generally exhibited increased Q 56 -YFP levels ( Fig. 4 ) and also aggregates with a fibrous pattern similar to Q 30 -YFP WT yeast ( Supplementary Fig. S10 ). Thus, while hsp104Δ and pho5Δ may be characterized by an altered aggregation pattern, other strains did not appear to be different in this respect. To confirm the status of Hsp104 in other knockout strains of Group I, western blots were performed. Hsp104 was not detectable in the hsp104Δ strain. The levels of Hsp104 were unchanged in the pho5Δ strain and only affected in sin3Δ ( Supplementary Fig. S11 ). As altered expression levels of Q 56 -YFP, an altered oligomerization state and altered aggregate morphology were only apparent for pho5Δ and hsp104Δ , these genes seem to modulate pica through similar mechanisms. Q56 interferes with septin ring formation The FACS data, the influence of genome copies and the annotated function of the hits derived from the genome-wide screen point to an involvement of the budding process and cellular division in the generation of the pica phenotype. We thus tested whether certain landmark events during the division process are reached in pica cells using green fluorescent protein (GFP)-tagged proteins, previously described to assemble into defined cellular structures [40] . To be able to separate the polyQ fluorescence signal from GFP, the chromophore in pQ0 and pQ56 was exchanged from eYFP to mCherry, yielding pQ0cherry and pQ56cherry. The phenotype was retained upon transformation of these constructs into the marker strains. We initially examined Tub1-GFP-expressing cells to investigate the spindle architecture during mitosis and its extension into the daughter cell [41] . After transformation with pQ56cherry, we observed slightly less cells with assembled tubulin structures compared with pQ0cherry ( Fig. 5a ). While extended spindles usually reach into the daughter cells in the presence of the non-toxic pQ0cherry construct, we found apparently misshaped, bent spindles to appear in pica cells. 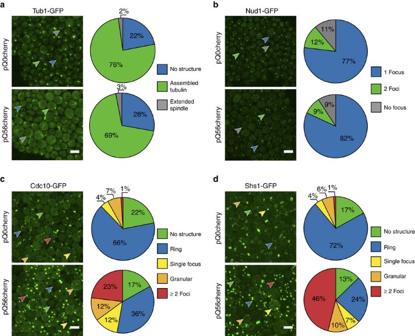Figure 5: pQ56 interferes with specific cellular structures. Fluorescent reporter strains were transformed with cytostatic and non-cytostatic polyQ constructs and the effect on reporter structures was examined. The arrowheads point to cells representative for a certain localization pattern and coloured according to their class for which the averaged quantiation result from three independent biological replicates is visualized in the pie chart to the right of each micrograph (Supplementary Fig. S13for corresponding bar charts, indicating error margins). The scale bar represents 5 μm in all panels. (a) Tub1-GFP is a marker for the spindle and only minor changes in the amount of cells with assembled tubulin structures can be detected. However, elongated spindles are slightly more frequent in pQ56cherry transformants and never extend into a bud or daughter. (b) Spindle pole bodies, labelled with Nud1-GFP may exhibit no, a single focal, or two focal depositions. They seem unaffected by pQ56cherry (c) Cdc10-GFP localizes to the septin ring, but also may be found not localized to a specific structure or exhibit granular or focal appearance to a low extent. When pQ56cherry is present, ring association is found less frequently, being substituted by an increased amount of granular or multifocal localization. (d) The effect observed for Cdc10-GFP is even more pronounced for the septin Shs1. Upon transformation with pQ56cherry ring association is substituted by a majority of cells exhibiting multifocal deposition of the septin. Figure 5: pQ56 interferes with specific cellular structures. Fluorescent reporter strains were transformed with cytostatic and non-cytostatic polyQ constructs and the effect on reporter structures was examined. The arrowheads point to cells representative for a certain localization pattern and coloured according to their class for which the averaged quantiation result from three independent biological replicates is visualized in the pie chart to the right of each micrograph ( Supplementary Fig. S13 for corresponding bar charts, indicating error margins). The scale bar represents 5 μm in all panels. ( a ) Tub1-GFP is a marker for the spindle and only minor changes in the amount of cells with assembled tubulin structures can be detected. However, elongated spindles are slightly more frequent in pQ56cherry transformants and never extend into a bud or daughter. ( b ) Spindle pole bodies, labelled with Nud1-GFP may exhibit no, a single focal, or two focal depositions. They seem unaffected by pQ56cherry ( c ) Cdc10-GFP localizes to the septin ring, but also may be found not localized to a specific structure or exhibit granular or focal appearance to a low extent. When pQ56cherry is present, ring association is found less frequently, being substituted by an increased amount of granular or multifocal localization. ( d ) The effect observed for Cdc10-GFP is even more pronounced for the septin Shs1. Upon transformation with pQ56cherry ring association is substituted by a majority of cells exhibiting multifocal deposition of the septin. Full size image We aimed to identify potential reasons for the spindle misorientations. The spindle pole body (SPB) is the organizational centre of the spindle. Nud1 is a component of the SPB outer plaque and in consequence an indicator for the status of the SPB. The SPB duplicates in S-phase and migrates to opposite poles of the nucleus during G2 phase. If cells were halted in late G2 phase or early mitosis before metaphase, an increased number of individual cells exhibiting two SPBs should become apparent. Microscopy of Nud1-GFP cells however did not point to a marked enrichment of cells bearing duplicate SPBs or potential severe mislocalization of SPB components ( Fig. 5b ), implying, that no defect is present in early mitosis. As a very early event during the budding and division process, the septin ring assembles in late G1 phase [42] . Septin ring formation is one of the initial events in the preparation of a mitotic event and is only disassembled after cytokinesis. The ring consists of septins, such as Cdc10. Cdc10-GFP localizes to this structure, allowing the detection of proper assembly of the ring. Cells transformed with non-toxic control plasmids exhibited mostly ring structures or no fluorescent structure ( Fig. 5c ). This situation changed markedly, when Q 56 -mCherry was present. Now, only one third of cells exhibited proper ring formation. The amount of cells with obviously abnormal foci rose from 1 to 23%. The effect of septin mislocalization became even more pronounced, examining Shs1-GFP, another septin homologue: Shs1-GFP was localized in rings or half-rings in 72% of cells transformed with the non-toxic control. However, in pica colonies from pQ56cherry plates, Shs1-GFP ring organization was drastically compromised ( Fig 5d ). Only 24% of cells were able to form a septin ring. The amount of cells bearing two or more focal deposits of Shs1-GFP rose from 1 to 46% with a third of these cells bearing more than four Shs1-GFP foci. The fact that around half of all yeast cells suffer from the mislocalization of septins suggests a defined point of growth inhibition during the yeast cell cycle. The strong reduction of correctly assembled rings implies that in particular the assembly or organization of the septin ring is hardly possible in the presence of extended polyQ stretches. We aimed at testing whether this disturbance was ameliorated in yeast cells resistant to the pQ56-induced toxicity. We thus analysed several weakly fluorescent, large colonies from Cdc10-GFP-tagged cells transformed with pQ56 and also from colonies grown on 4 mM GdnHCl plates. In all colonies analysed, the assembly of Cdc10 into the septin ring reverted to normal with respect to cells with focal depositions ( Table 1 ). The data indicate that pica is not caused by direct interference with the mitotic process itself, but rather by disturbing the formation of a functional septin ring structure. The reversion to normal ring assembly and the concomitant loss of pica by GdnHCl treatment or hyperploidization highlight that these effects can be cured by resistance-generating mechanisms. Table 1 Survivor colonies and growth on GdnHCl abolish the effect of polyQ proteins on septins. Full size table In this study, we describe a polyQ aggregation system, mimicking toxicity by strongly inhibiting the growth of S. cerevisiae . Such pica colonies are characterized by enlarged cells and a fraction of cells with a non-haploid amount of genome copies (2 N /4 N ). We aimed to map the point of interference with the yeast cell cycle and uncover pQ 56 -YFP-specific effects on two structures important to the budding process. The experimental data indicate that extended spindles fail to reach into daughter cells, when pQ56 is present, implying a dysregulation of the spindle extension process. We also see a striking failure to assemble correct septin rings. However, the appearance of additional (up to 10) focal deposits of the septins Shs1 and Cdc10 may suggest, that cells are able to select the bud site but not to rearrange the septins as required for the maturation of the ring geometry, which in turn is a prerequisite for bud formation [43] . We thus assume that pQ 56 -YFP interferes with bud formation and mainly causes pica by affecting this pathway. Extended metaphase/anaphase spindles that do not reach into daughters may result from a leakiness of the morphogenesis checkpoint, which usually delays the cell cycle, when septin assembly is compromised [42] . It is interesting that recently a cell cycle arrest by the overexpression of the prion RNQ1 has been documented [44] . This effect arose from the specific sequestration of a SPB component, leading to the activation of the Mad2 checkpoint and endoreduplication events. Our data suggest that the interference with septin assembly is possibly another mechanism of cell cycle delay by aggregation prone proteins, inducing an increased number of polyploid cells by endoreduplication in the pica population. Notably, in the system presented here, yeast cells containing more than a haploid chromosome set are resistant to pica ( Fig. 6 ). We also encounter similar growth-promoting conversions for spontaneous survivor colonies after transformation of haploid cells with pQ56, but their incidence is low. For a Huntington’s disease mouse model, data are controversial, whether aneuploid or hyperploid fibroblasts are more frequent in mice transgenic for Htt150Q [45] , [46] . 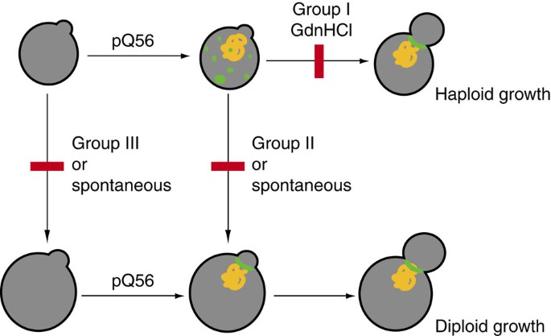Figure 6: A model for the development of and the escape frompica. Thepicaphenotype is generated by the expression and presumable aggregation of Q56-YFP (yellow) and the subsequent inability of cells to follow the normal haploid growth cycle, potentially caused by compromised septin deposition (green). Deletion of Group I genes and treatment with GdnHCl restores growth as haploid yeast cells and septin ring assembly. An alternative route is switching to diploid growth, which under normal conditions is blocked by Group II (and Group III) genes. This switching event happens for Group II genes only in response to the cytostatic pressure from Q56-YFP. In deletion strains for Group III genes, this switching to 2Nstates happens also under control conditions, leading to constitutive cycling at higher ploidy and resistance topica,as well as a restored capability to assemble septin rings. Figure 6: A model for the development of and the escape from pica . The pica phenotype is generated by the expression and presumable aggregation of Q 56 -YFP (yellow) and the subsequent inability of cells to follow the normal haploid growth cycle, potentially caused by compromised septin deposition (green). Deletion of Group I genes and treatment with GdnHCl restores growth as haploid yeast cells and septin ring assembly. An alternative route is switching to diploid growth, which under normal conditions is blocked by Group II (and Group III) genes. This switching event happens for Group II genes only in response to the cytostatic pressure from Q 56 -YFP. In deletion strains for Group III genes, this switching to 2 N states happens also under control conditions, leading to constitutive cycling at higher ploidy and resistance to pica, as well as a restored capability to assemble septin rings. Full size image Using the yeast deletion library, we identify three groups of genes, which are required to obtain the pica phenotype. The deletion of these genes leads to resistance against Q 56 -YFP-induced growth arrest ( Fig. 6 ). Surprisingly, the set of genes we uncover has only limited overlap with similar genome-wide approaches performed before. A screen on Htt toxicity only shares three genes we found in our screen ( HSP104 , BFR1, CYK3 ) [15] . Our screen only recovers four strains ( HSP104 , PHO5 , CYK3 , RAD6) of 58 knockout strains previously documented to be [ pin − ] in the mainly [ PIN + ] knockout library [47] . We find the largest overlap of hits ( hsp104Δ , spt4Δ , scp160Δ , bfr1Δ, swa2Δ and asc1Δ ) with a screen seeking deletions that reduce the inducibility of the [ PSI + ] phenotype [38] . However, the pQ56 system seems to be largely independent of the endogenous prion state, implying that the genes overlapping contribute to both, prion maintenance and substantiating the pica phenotype. Group I hits are able to rescue, preserving the haploid state. Most likely, in these strains the cytostatic species is abolished or its direct targets are modified to become insensitive to its mode of action. The first seems true for hsp104Δ and pho5Δ . Both strains behave highly similar in all assays and only hsp104Δ has been shown before to prevent aggregate toxicity [15] , [38] . The effect we observe upon the loss of Hsp104 is also surprising in the context with other studies that found this protein together with actin necessary for aggregate clearance from daughter cells [33] , [48] . This function of Hsp104 seems counterproductive to prevent pica in our experimental set-up. However, hyperploidy as a rescuing mechanism for pica is pronounced for other strains, retrieved in our screen. Albeit previously mainly haploid, Group II genes show an increased conversion to a diploid state in the presence of Q 56 -YFP, implying that the absence of Group II genes facilitates the accumulation of genome copies. Group III strains are polyploid also when transformed with control constructs and consequently by default resistant to pQ56-YFP. The uncovered genes are partly known to be involved in the control of ploidy (for example, SCP160 ), but others have not been related to this process yet. It is interesting that increased ploidy is also capable to generate resistance in HttQ103 transformed cells, although more subtly. This observation implies that ploidy as a mechanism of resistance is conserved for polyQ proteins, largely independent of the flanking sequences. How does polyploidy relate to resistance against pica ? We find that spontaneous survivor colonies are not defective in septin assembly. It may consequently be speculated that diploid cells have requirements different from haploid cells concerning the composition, the timepoint of assembly, or the geometry of the septin ring and consequently are insensitive to polyQ-induced cytostasis. While septin ring formation and the concerted action of actin networks and the Hsp104 system to retain aggregates in mother cells is a characteristic of fungal cells, there notably are potentially homologous metazoan processes and cellular structures: septins maintain dendritic spine individualization and are associated to neuropathological conditions [49] ; molecular filters based on actin at the axonal initial segment are responsible for retaining specific macromolecules in the soma of neurons [50] . Thus, during the maintenance of mammalian neuronal networks, cellular structures and control mechanisms similar to those found at the bud neck in yeast might be compromised by polyQ proteins. Yeast strains The haploid Saccharomyces Genome Deletion Project library (EUROSCARF, Frankfurt, Germany) in the BY4741 background ( MAT a ; his3 Δ 1 ; leu2 Δ 0 ; met15 Δ 0 ; ura3 Δ 0 ) was used for screening. Further, we employed the strains BY4742 ( MAT α), BY4743 ( MAT a /α) [51] , PY4994 ( MAT α/α), PY4995 ( MAT a / a ), PY5006 ( MAT a / a / a / a ) and PY5007 ( MAT α/α/α/α) [23] to study the influence of different mating types and ploidy on the development of pQ56-induced toxicity. To rule out false-positive strains among our hits due to MAT a /α genotype, all strains were tested four times for their mating type by PCR and removed from the gene list, if they were positive for both mating types ( Supplementary Table S2 ) in one experiment. The genotype of all other strains in the study was MAT a , even when di/hyperploid according FACS analysis, which is indicative of a MAT a / a or MAT a / a / a / a genotype. The knockout cassette was sequenced to confirm the identity of the knockout strains, uncovered in the screen. For the PHO5 knockout strain, also the locus of HSP104 was confirmed to correspond to the WT sequence, to rule out effects of single-site mutations in the coding sequence of this protein. For the analysis of cellular structures affected by the presence of polyQ proteins, the respective strains of the Yeast GFP fusion collection in the background of EY0986 ( MAT a ; his3Δ1 ; leu2Δ0 ; met15Δ0 ; ura3Δ0 ) were deployed [40] . Generation of the polyQ expression constructs Expression constructs were generated by fusing 0, 30 or 56 glutamine codons to the 5′ end of a polylinker upstream of the eYFP gene (Clontech, Mountain View, USA; see Supplementary Fig. S12 for sequence information). Coding sequences were synthesized by GeneArt AG (Regensburg, Germany) and subcloned into the plasmid p425GPD [52] , resulting in pQ0, pQ30 and pQ56. pQ0cherry and pQ56cherry were obtained by ligating a BstAPI/SalI (New England Biolabs, Frankfurt, Germany) fragment encoding the chromophoric protein into the accordingly digested pQ0 and pQ56 vectors, preserving the polyQ and polylinker regions. All constructs were prepared on a midiprep scale (Promega, Fitchburg, USA) and sequenced to rule out polyQ shortening or construct mixtures. Yeast growth and transformation Transformations were performed using a simplified LiOAc method. Cells were grown in YPD medium (Carl Roth, Karlsruhe, Germany) for 48 h at 30 °C. Per transformation 200 μl of culture were sedimented for 10 min at 2,500 g . Cells were resuspended in 150 μl of a solution containing 40% (w/v) PEG4000, 100 mM LiOAc, 10 mM TRIS/HCl (pH 7.5), 1 mM EDTA, 5.1 μg ml −1 salmon carrier DNA (Sigma-Alrich, St Louis, USA), 0.4 mM dithiothreitol (final concentrations) and 100 ng of plasmid DNA. Cells were incubated in this solution for 16 h at room temperature. The mixtures were heat shocked for 1 h at 42 °C. The transformants were plated on the appropriate supplemented minimal medium containing either 2% glucose for constitutive plasmids or the same amount of galactose for inducible plasmids. The same procedure was applied to transform the knockout strains in 96-well plates. For screening, strains were grown separately in deep-well plates in 600 μl of YPD. Cultures were scored after 4 days of incubation at 30 °C. About 2 × 10 3 homogeneously growing colonies were normally observed per plate, if non-toxic constructs were transformed. For analysis of yeast viability 10 4 cells were replated on the appropriate supplemented minimal medium agar and the number of CFU scored after 4 days of incubation at 30 °C. Prion curing of yeast strains was performed by triplicate sequential passage on YPD, containing 4 mM GdnHCl. Each passage was incubated for 2 days. Analysis of cell size by microscopy Yeast cells were analysed by standard light microscopy. Colonies were picked from plates and resuspended in 100 μl of CSM solution and transferred to agar pads for differential interference contrast microscopy (DIC) on a Zeiss Axiovert 200 microscope (Zeiss Biomedical, Oberkochen, Germany). To obtain the cellular cross-sectional area, cells were fixated in 70% ethanol. The solution was immediately supplied with an equal volume of 0.1% methylene blue (Sigma-Aldrich, St Louis, USA) to obtain high contrast. Images were recorded on an Axiovert 200 (Zeiss Biomedical, Oberkochen, Germany) in bright field mode. Using ImageJ, the images were thresholded to obtain black and white representations. Deploying the particle analysis plug-in of ImageJ, the cells were picked and cross-sectional areas measured. Cells out of focus or touching the image border were excluded from analysis. Fluorescence microscopy For low magnification fluorescence microscopy of yeast colonies a Leica MZ16-FA (Leica, Wetzlar, Germany) stereo microscope was used. For high resolution microscopy of individual yeast cells, an Axiovert 200 microscope (Zeiss Biomedical, Oberkochen, Germany) and the appropriate filter set for YFP fluorescence and DIC for transmitted light were deployed. Confocal microscopy was performed on a Leica SP5 laser scanning microscope. YFP and GFP were excited, using the 514 nm and 458 nm lines of an Argon laser at 6% total laser power, respectively. mCherry was imaged using the 543 nm line of a HeNe laser at 30% of the emitted intensity. Gain and offset were adjusted to exploit the dynamic range of the photomultipliers, but remained unchanged among different samples of each co-localization strain to ensure comparable intensities. If necessary, linear adaptation of contrast and brightness and were performed using ImageJ. Flow Cytometry FACS was performed on a BD FACSCalibur Flow Cytometer (Becton Dickinson, Heidelberg, Germany). Yeast cells were transformed, plated and incubated for 4 days as described above. To enable analysis of the dominant colony population, large colonies were removed from pQ56 transformed plates. Plates were washed with 100 mM TRIS/HCl (pH 7.5), 50 mM NaCl and yeast cells were collected. Cells were fixated over night using 70% ethanol and then resuspended in 50 mM Na-Citrate (pH 7), followed by sonication in a waterbath for 30 s. Cell densities were normalized to be 10 7 cells ml −1 . Cells were treated over night with 0.25 mg ml −1 boiled RNAse A at 37 °C and for 2 h at 50 °C with 1 mg ml −1 Proteinase K (both Sigma-Aldrich, St Louis, USA). Yeast were stained with propidium iodide (Sigma-Aldrich, St Louis, USA) at a concentration of 20 μg ml −1 . Cells were sonicated as above and thoroughly resuspended right before FACS analysis. To exclude cell doublets or cellular debris from analysis, events were gated accordingly. For most strains, histograms were acquired in linear mode and measurements were repeated in log mode, if cells exhibited states of ploidy >4 N . All histograms were normalized to the fluorescence intensity of the 1 N peak of strain BY4741. Native agarose gel electrophoresis Native agarose gel electrophoresis was performed for the analysis of the oligomerization properties [39] . To this end, cells were harvested as described for FACS analysis and resuspended in a buffer containing 100 mM Tris/HCl (pH 7.5), 50 mM NaCl, 10 mM β-ME, protease inhibitor cocktail FY (1:25 dilution, Serva, Heidelberg, Germany). Mechanical disruption of 450 μl of cell suspension was achieved by adding 900 mg of 0.25–0.50 mm glass beads (Carl Roth, Karlsruhe, Germany) and subsequent shaking at 4 °C in 4 pulses of 2 min at 30 Hz in a MM400 bead mill (Retsch, Haan, Germany). The disruption efficiency was >90% of all cells, as verified by phase contrast microscopy on an Axiovert 200 microscope (Zeiss Biomedical, Oberkochen, Germany). Lysates were kept at 4 °C and normalized by Bradford assay (Serva, Heidelberg, Germany). After being supplied with 5 × loading buffer (32 mM TRIS/HCl pH 8.3, 50% glycerol, 0.1% bromphenol blue), 30 μl of sample were loaded onto 1% agarose gels in running buffer (190 mM glycine, 25 mM Tris, pH 8.3). Electrophoresis was carried out at a potential of 3 V cm −1 of gel length for 17 h at 4 °C. Detection of the polyQ protein occurred via the eYFP moiety using the appropriate settings on a Typhoon 9200 multimode imager (GE Healthcare, Munich, Germany). Western Blot For western blots, yeast lysates were prepared and normalized as described for native agarose gel electrophoresis. Lysates were supplemented with 5 × Laemmli-buffer and subjected to SDS–polyacrylamide gel electrophoresis using ServaGel neutral pH 7.4 gradient gels (Serva, Heidelberg, Germany). Gels were electroblotted semi-dry onto polyvinylidene difluoride membranes (Carl Roth, Karlsruhe, Germany). Blots were probed with goat anti-GFP (1:5,000, Rockland, Gilbertsville, USA) and anti-Hsp104 (1:40,000) antibodies raised in rabbit. As loading controls, anti-Hsp82 (1:80,000) antibody raised in rabbit and mouse anti-PGK (1:15,000, Life Technologies, Darmstadt, Germany) were used. Detection was carried out using secondary peroxidase conjugated antibodies against mouse, rabbit and goat (Sigma-Aldrich, St Louis, USA) and the ECL detection kit (GE Healthcare, Munich, Germany), all according to the manufacturer's instructions. Interaction network To generate an interaction network, gene identifiers were uploaded to the string database ( http://string-db.org , version 9.0) [53] . The obtained interaction network was further layouted using Cytoscape (version 2.7.0, http://www.cytoscape.org ) [54] . Grouping according to biological function was performed according to literature cited in the main text and gene annotation in the Saccharomyces Genome Database ( http://www.yeastgenome.org ). How to cite this article: Kaiser, C.J.O. et al . A network of genes connects polyglutamine toxicity to ploidy control in yeast. Nat. Commun. 4:1571 doi: 10.1038/ncomms2575 (2013).